Identifying sources of tick blood meals using unidentified tandem mass spectral libraries Rapid and reliable identification of the vertebrate species on which a disease vector previously parasitized is imperative to study ecological factors that affect pathogen distribution and can aid the development of public health programs. Here we describe a proteome profiling technique designed to identify the source of blood meals of haematophagous arthropods. This method employs direct spectral matching and thus does not require a priori knowledge of any genetic or protein sequence information. Using this technology, we detect remnants of blood in blacklegged ticks ( Ixodes scapularis ) and correctly determine the vertebrate species from which the blood was derived, even 6 months after the tick had fed. This biological fingerprinting methodology is sensitive, fast, cost-effective and can potentially be adapted for other biological and medical applications when existing genome-based methods are impractical or ineffective. Trophic relationships are primary determinants of both population dynamics and the distribution and abundance of organisms [1] , [2] , [3] . For example, the distribution and abundance of potential host species of parasites, as well as the quality of those host species, have a dominant influence on the population densities and geographic ranges of parasites [1] , [4] , [5] . Although the distribution and abundance of parasites are important to human health and economics [6] , [7] , little is known about the extent to which different vertebrate species affect the dynamics of most parasite species. Many haematophagous parasites also vector microbial pathogens that are the primary cause of emerging infectious diseases [8] . Further, human disease risk is often correlated with the distribution and abundance of these disease vectors [9] , [10] , [11] , [12] . Ixodes scapularis ticks are of particular public health importance as they are a common vector of several emerging infectious diseases in the eastern United States including anaplasmosis, babesiosis and Lyme disease [13] . The natural ecologies of many vectors remain obscure because of the inherent difficulties in collecting the quantitative data necessary to assess the relevance of each host species to parasite population dynamics [5] , [14] , [15] , [16] , [17] , [18] . Traditionally, labour-intensive quantification of the parasite burden on all potential wildlife species was needed [19] , [20] . These data are often heavily biased by the variation in trapping success among animal species [5] , [16] . Analysis of the vertebrate blood remaining in haematophagous insects is an alternative and highly sought-after method to determine the importance of each species to the parasite population [21] , [22] , [23] , [24] , [25] , [26] . Identification of the source of the blood found in vectors that are seeking a subsequent host is also considerably less labour intensive than observing vectors on live vertebrates. Moreover, collections of host-seeking vectors, as opposed to vectors collected from wildlife hosts, provide a random sample resulting in an unbiased quantification of the frequency in which each host species is parasitized. Current methodologies employed to identify previous blood meals, including serological techniques [22] , [23] , [25] , DNA-based methods [21] , [24] and protein analysis [26] , [27] , confront at least one of the hurdles that prevent their practical use. First, remnants of blood from previous hosts are often severely degraded when vectors begin seeking another host, drastically reducing the efficacy of most procedures [21] , [28] , [29] , [30] , [31] , [32] , [33] , [34] . Second, all methods to date select one or several target molecules a priori to distinguish among a set of a priori- selected host species. Random degradation or digestion of the target molecules limits the success of these methodologies even though non-target molecules that can distinguish among host species may still be present [26] , [32] . Further, target molecules may be identical among host species that are not included in a study, thus reducing confidence in these procedures. Most importantly, suitable target molecules have not been characterized in the majority of wildlife species, thus limiting these methods to well-characterized model organisms. In summary, a robust, universal method to analyse vector blood meals is needed to identify the impact of host species on the ecology and epidemiology of disease vectors. In the present study, we describe a non-targeted, genome-free, proteomics-based, spectral-matching [35] , [36] , [37] , [38] , [39] , [40] methodology designed to identify the source of blood meal remnants in haematophagous arthropods. This methodology can be used to determine the ecological importance of each species in a vertebrate community to the maintenance of populations of haematophagous arthropods. We empirically validated this methodology by identifying the source of blood remnants in blacklegged ticks ( I. scapularis ) that had fed on different vertebrate species. Remnants of blood in the ticks can be detected and correctly classified to the vertebrate species in the majority of cases, even for ticks that had completed a moult and were active for up to 6 months since their last blood meal. Construction of spectral libraries Whole blood from 24 vertebrate species were individually trypsin-digested and analysed by liquid chromatography–tandem mass spectrometry (LC-MS 2 ). Reference libraries were built for each species using SpectraST (version 4.0), which was adapted to build spectral libraries from unidentified spectra ( Fig. 1 ). Spectra that are highly similar and therefore likely derived from identical peptides were detected by similarity clustering and merged into higher-quality consensus spectra ( Supplementary Methods ). Unlike conventional spectral libraries, similarity clustering is necessary for consensus spectrum building when peptide identifications are not known. Collectively, the spectral libraries contained 9,045 consensus spectra, 1,039 (11.5%) of which were detected in multiple species. The distribution and relative abundance of spectra among vertebrate species are visually represented in Fig. 2 . Spectra from the blood of M. musculus , the only species for which a genome sequence database is available and peptide identifications could be made reliably, were identified by conventional sequence searching to reveal the underlying protein distribution of the spectral libraries ( Fig. 3 ). 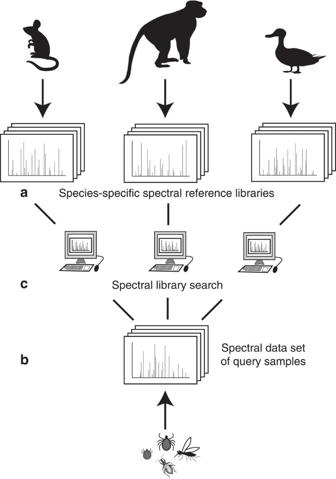Figure 1: A schematic overview of blood meal identification using spectral proteomes. (a) Species-specific spectral reference libraries are built from LC-MS2analyses of trypsin-digested whole blood from potential host vertebrates. Spectra do not require peptide identifications as long as they are reproducible. (b) Collection of query LC-MS2spectral data sets obtained from vectors days to months after blood feeding. Query spectral data sets include the vector proteome and the proteome of the remnants of blood from the previous blood meal. (c) Similarities between the spectral data set and each spectral reference library are determined using a Spectral Data set Similarity Scoring (SDSS) algorithm. The SDSS algorithm provides a quantitative similarity measure between sets of spectra, and hence the proteomes underlying the data sets, using the number of query spectra that matched each reference library spectrum. Figure 1: A schematic overview of blood meal identification using spectral proteomes. ( a ) Species-specific spectral reference libraries are built from LC-MS 2 analyses of trypsin-digested whole blood from potential host vertebrates. Spectra do not require peptide identifications as long as they are reproducible. ( b ) Collection of query LC-MS 2 spectral data sets obtained from vectors days to months after blood feeding. Query spectral data sets include the vector proteome and the proteome of the remnants of blood from the previous blood meal. ( c ) Similarities between the spectral data set and each spectral reference library are determined using a Spectral Data set Similarity Scoring (SDSS) algorithm. The SDSS algorithm provides a quantitative similarity measure between sets of spectra, and hence the proteomes underlying the data sets, using the number of query spectra that matched each reference library spectrum. 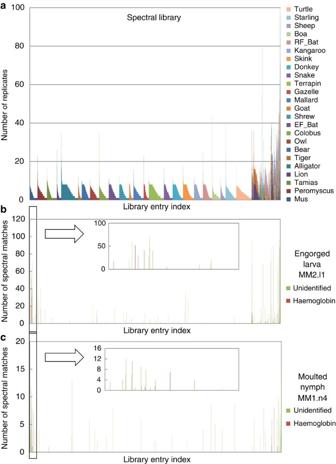Figure 2: Reference spectral libraries of the blood proteomes of 24 vertebrate species. (a) The diversity and abundance of unique and shared spectra in the spectral reference libraries visualized as a bar chart. Each bar along the abscissa represents a distinct consensus spectrum, and the height of the bar represents the number of replicates merged into that consensus. Bars are color-coded to represent the species from which the replicates originate. The multi-colored bars to the right represent spectra that are observed in multiple species. Example of spectral data set matches for (b) one larva engorged withM. musculus(MM2.l1) or (c) one moulted nymph held at 25 °C for 6 months after feeding onM. musculus(MM1.n4). The majority of spectral matches for the tick data sets are to library spectra from the correct species (M. musculus), or to spectra from multiple species includingM. musculus. The matched spectra are subjected to sequence searching against haemoglobin sequences. Although some spectral matches are due to haemoglobin (red), many other matches cannot be identified by sequence searching (green). Full size image Figure 2: Reference spectral libraries of the blood proteomes of 24 vertebrate species. ( a ) The diversity and abundance of unique and shared spectra in the spectral reference libraries visualized as a bar chart. Each bar along the abscissa represents a distinct consensus spectrum, and the height of the bar represents the number of replicates merged into that consensus. Bars are color-coded to represent the species from which the replicates originate. The multi-colored bars to the right represent spectra that are observed in multiple species. Example of spectral data set matches for ( b ) one larva engorged with M. musculus (MM2.l1) or ( c ) one moulted nymph held at 25 °C for 6 months after feeding on M. musculus (MM1.n4). The majority of spectral matches for the tick data sets are to library spectra from the correct species ( M. musculus ), or to spectra from multiple species including M. musculus . The matched spectra are subjected to sequence searching against haemoglobin sequences. Although some spectral matches are due to haemoglobin (red), many other matches cannot be identified by sequence searching (green). 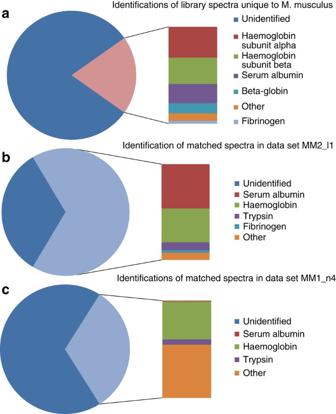Figure 3: Underlying protein distribution of the blood proteome ofM. musculus. Peptide identifications of spectra used to build or search theM. musculuslibrary by sequence searching. (a) The protein distribution of the identifications of the library spectra unique toM. musculus. (b,c) The protein distributions of identifications of spectra matched to theM. musculuslibrary for two data sets: MM1.n4 (a moulted nymphal tick) and MM2.l1 (an engorged larva), respectively. A large fraction of spectra remain unidentified by sequence searching, despite the comprehensiveness of theM. musculusprotein sequence database. Among identified spectra, subunits α and β of haemoglobin, serum albumin, β-globin and fibrinogen are the most frequent protein identifications found. Full size image Figure 3: Underlying protein distribution of the blood proteome of M. musculus . Peptide identifications of spectra used to build or search the M. musculus library by sequence searching. ( a ) The protein distribution of the identifications of the library spectra unique to M. musculus . ( b , c ) The protein distributions of identifications of spectra matched to the M. musculus library for two data sets: MM1.n4 (a moulted nymphal tick) and MM2.l1 (an engorged larva), respectively. A large fraction of spectra remain unidentified by sequence searching, despite the comprehensiveness of the M. musculus protein sequence database. Among identified spectra, subunits α and β of haemoglobin, serum albumin, β-globin and fibrinogen are the most frequent protein identifications found. Full size image Accuracy of clustering algorithm The performance of the clustering algorithm was validated by comparing a spectral library built by similarity clustering without knowledge of peptide identifications, as described above, and a spectral library built from sequence-search results of the same data. The latter is possible for species with comprehensive and high-quality sequence databases such as M. musculus . We implemented this strategy on a larger data set containing 40 runs of a SDS–PAGE-fractionated protein digest sample of M. musculus blood. In this data set, 20,156 of the 38,010 acquired tandem mass spectra survived the spectrum filter and were similarity-clustered, as described above, into 3,584 clusters. At the same time, traditional sequence searching ( Supplementary Methods ) identified 10,324 spectra from the same data set to a total of 1,566 distinct identifications (44% of 3,584). Therefore, less than half of all clusters were identified by sequence searching, likely because of incomplete search space (for example, due to modifications not considered) and insufficient discriminating power of sequence searching. Of the clusters with at least one originating replicate identified, 1,492 entries (95%) are ‘pure’ clusters with only one sequence identification, 29 (2%) entries are ‘mixed’ ones with two or more different identifications, 35 (2%) entries are ‘split’ clusters, for which the same identification was also found in another cluster, and 10 entries (1%) are both ‘mixed’ and ‘split’ ( Fig. 4 ). This result suggests that the clustering algorithm is largely capable of merging spectra that originate from the same peptide, but not those that originate from different peptides. 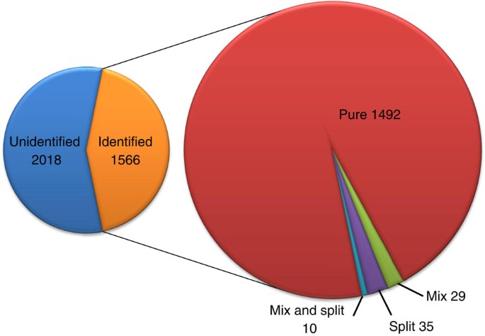Figure 4: Correspondence between spectrum clusters and sequence-search results. The clustering algorithm is validated using a much largerM. musculusfractionated blood data set. Among the 1,566 clusters that have at least one spectrum identified by SEQUEST, an overwhelming number (1492/1566=95%) of them are ‘pure’ clusters that have a single and unique peptide identification inM. musculusnot found in any other cluster. Figure 4: Correspondence between spectrum clusters and sequence-search results. The clustering algorithm is validated using a much larger M. musculus fractionated blood data set. Among the 1,566 clusters that have at least one spectrum identified by SEQUEST, an overwhelming number (1492/1566=95%) of them are ‘pure’ clusters that have a single and unique peptide identification in M. musculus not found in any other cluster. Full size image Identification of blood meal source in engorged larvae The correct vertebrate species was identified as the source of the blood meal in all but one engorged larvae tested, demonstrating proof-of-principle evidence of the efficacy of this methodology ( Table 1 ). The identification is made by finding the reference library with the highest similarity to the spectral data set of the blood meal to be tested. A spectral data set similarity score (SDSS) developed for this application provides a quantitative similarity measure between two spectral data sets, and hence the entire proteomes underlying the data sets. Using this algorithm, the blood in all five of the larval ticks that had fed to repletion on either of a two M. musculus mice was determined to be most similar to the M. musculus spectral reference library. These results had high bootstrap support (>99%), indicating that a large number and wide variety of spectra are available to correctly identify the blood in these ticks as M. musculus blood ( Table 1 ). An example spectral data set match is shown in Fig. 2 . These data also demonstrate that the presence of vector proteins in the sample do not detract from the ability of this methodology to identify the source of the blood meal. Correct identifications were also achieved for all larval ticks that had fed on any of the four Peromyscus leucopus mice or any of the three Tamias striatus chipmunks, all with high bootstrap support (>99%) ( Table 1 ). Interestingly, the blood in the larval ticks that had fed on two of the three Sciurus carolinensis squirrels was not identified as squirrel blood, as there was no squirrel blood spectral reference library, but instead matched most closely with the chipmunk spectral reference library ( Table 1 ), the species that is evolutionarily most closely related to S. carolinensis among the reference libraries. Thus, this method can also identify an unknown sample to the closest-related species represented in the spectral libraries. This finding is corroborated by the evolutionary accuracy of the phylogenies built from the spectral reference libraries discussed below. Table 1 The species on which an engorged larva ( I. scapularis ) previously parasitized can be confidently determined through proteome profiling. Full size table A recent publication reported the protein sequences of haemoglobin subunits of several vertebrate species by de novo sequencing and suggested that these sequences can be used to identify the source of blood meals in vectors [27] . To benchmark the methodology presented here, we also searched the proteomic data from our ticks against the haemoglobin sequences of M. musculus , P. leucopus and T. striatus by sequence database searching. Identification of the source of the blood meal from engorged larval ticks was also effective using methods based on detecting haemoglobins by sequence searching algorithms ( Supplementary Table S1 ). Similar to the results by our method, larval ticks that had fed upon S. carolinensis could also be identified as ticks that had fed upon T. striatus if S. carolinensis haemoglobin sequences are not included in the database. Identification of the blood meal in moulted nymphal ticks In 23 of the 26 cases, the spectral data sets derived from the remnants of blood in moulted nymphal ticks were identified to the spectral reference libraries of the species on which the tick had fed as a larva ( Table 2 , Fig. 2 ). Of the ticks that fed on M. musculus, the M. musculus spectral library was the most similar for all of the nymphs that were held at 25 °C for 1 month (6/6) and for 3 months (6/6) after blood meal, while the M. musculus spectral library was the most similar for the data sets from 4 of 6 nymphs held at 25 °C for 6 months before analyses. The statistical confidence in M. musculus as the source of the previous blood meal was >76% (bootstrap support) for each of the correctly classified nymphs. The two data sets that were not identified to the M. musculus were not misidentified to another organism; they simply had very low similarity scores with all spectral libraries, suggesting that little MS 2 data from the blood proteome was collected. More importantly, the spectral data sets from seven of eight nymphal ticks that had fed as larvae on natural reservoir hosts ( P. leucopus (5/6) and T. striatus (2/2)) and subsequently held at 25 °C for 5 months were successfully identified to the animal on which the ticks had previously fed, each with high bootstrap support ( Table 2 ). These data strongly support the utility of the spectral matching methodology to identify the source of previous blood meals in nymphal ticks that are collected in nature. Table 2 The species on which moulted nymphs ( I. scapularis ) parasitized during their larval stage can be confidently determined. Full size table Identification of the source of the blood meal from moulted nymphal ticks was less effective when peptide identification relied upon de novo sequenced haemoglobin subunits ( Supplementary Table S2 ). There were no instances in which the traditional sequence-based peptide identification methodology correctly identified the source of a blood meal that could not be identified using the spectral searching algorithm. Furthermore, the sequence-based method failed to identify the source of the blood meal for two ticks that fed on lab mouse, 4 out of 6 ticks that had fed on a white-footed mouse, and both ticks that had fed on a chipmunk. In these tick samples, no confident identification to any haemoglobin sequences were found. These results indicate that relying on a priori- selected target proteins (haemoglobin-α and -β) for identification was more prone to failure than the spectral matching algorithm described when the blood meal has undergone digestion over time. This is likely because the target proteins may have been degraded, whereas our proteome profiling strategy is still able to identify the source of the blood meal based on spectra from other, non-target, proteins. Although haemoglobin is the most abundant protein in vertebrate blood, only a small fraction of the matching spectra utilized by our method can be identified to haemoglobin sequences ( Figs 2 and 3 ). Multiple blood sources Although I. scapularis ticks feed only once per life stage, other arthropod vectors feed multiple times in rapid succession, which could hinder the identification of one or more sources of the blood in the vector. The ability to correctly identify the source of blood from vectors that had fed multiple times using the spectral matching methodology presented here was determined by experimentally mixing whole blood from different species at specified ratios. Whole blood from an African lion ( Panthera leo ) was mixed with blood from either an Amur tiger ( Panthera tigris ), an American alligator ( Alligator mississippiensis ) or a red kangaroo ( Macropus rufus ) at lion: other ratios of 1:1, 1:5 or 1:10. The choice of species was determined by the evolutionary relatedness ranging from very related to distantly related. Proteins from mixed blood samples were analysed by liquid chromatography - tandem mass spectrometry (LC-MS 2 ) and the SDSS algorithm as described above. The spectral matching methodology can successfully identify one of the two true species in all cases (with high bootstrap support), even if blood from both species is roughly at equal concentrations ( Fig. 5 ). In addition, when one source of blood is at much greater concentrations than the other (ratios of 1:5 and 1:10), the more concentrated source is identified as the top-scoring hit in all cases, while the SDSS for the less-abundant source varies. It is likely that blood derived from one of the multiple feedings will be predominant in a vector because of digestion between feedings or differences in the amount of blood acquired from each host. Under this scenario, this source of blood is likely to be identified by this method, despite contamination with other blood sources. Although the source of the blood making up the minor fraction can potentially be identified when it is at relatively high concentrations, a more sophisticated statistical method, as well as experimental samples that have fed on multiple host species, is needed to properly assess the validity of this method in identifying blood mixtures. Nevertheless, one of the true sources of the blood in a vector that has taken two blood meals in rapid succession can be identified with high confidence. 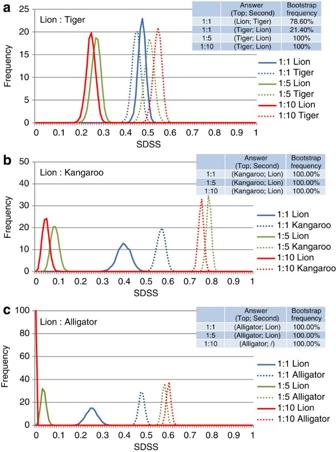Figure 5: Identifying mixed blood samples. The score histograms of matches to spectral libraries of lion (solid lines) and the other animal (dashed lines) are shown for three different mixing ratios (lion: other)—blue 1:1 green 1:5 and red 1:10 for (a) mix of lion and tiger blood, (b) mix of lion and kangaroo blood and (c) mix of lion and alligator blood, respectively. These mixed blood data sets matched the spectral libraries of all other spectral libraries with very low scores (<0.01). The species with the highest score and the second highest scores, together with the bootstrap frequencies of the highest-scoring identification, are shown in the inset tables. Figure 5: Identifying mixed blood samples. The score histograms of matches to spectral libraries of lion (solid lines) and the other animal (dashed lines) are shown for three different mixing ratios (lion: other)—blue 1:1 green 1:5 and red 1:10 for ( a ) mix of lion and tiger blood, ( b ) mix of lion and kangaroo blood and ( c ) mix of lion and alligator blood, respectively. These mixed blood data sets matched the spectral libraries of all other spectral libraries with very low scores (<0.01). The species with the highest score and the second highest scores, together with the bootstrap frequencies of the highest-scoring identification, are shown in the inset tables. Full size image Blood proteome divergence is evolutionary conserved Bayesian phylogenies derived from the presence or absence of each spectrum in each spectral reference library suggest that the degree of similarity in spectral libraries derived from blood proteomes is correlated with evolutionary relatedness. Bayesian phylogenies constructed using evolutionary models designed for restriction digest data resulted in topologies that recapitulate the known relationships among the vertebrate species ( Fig. 6 ). All nodes in the phylogeny constructed using the variable evolutionary model in MrBayes were supported by the data. The choice of evolutionary model for phylogenetic reconstruction did not affect the relationships among species, although branch lengths differed and posterior support for nodes was generally lower (data not shown). 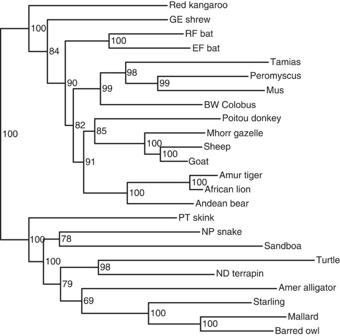Figure 6: Evolutionary relationships are accurately resolved from blood proteomes. Bayesian phylogenies constructed in MrBayes using the presence or absence of each spectrum in each reference library in thevariableevolutionary model designed for restriction digest data resulted in a phylogeny that recapitulates the established relationships among these species. Figure 6: Evolutionary relationships are accurately resolved from blood proteomes. Bayesian phylogenies constructed in MrBayes using the presence or absence of each spectrum in each reference library in the variable evolutionary model designed for restriction digest data resulted in a phylogeny that recapitulates the established relationships among these species. Full size image Evolutionary resolution of the spectral matching methodology The level of biological organization (species, population or individual) that can be distinguished using the proposed methodology was investigated using spectral data derived from whole blood. To allow for separate reference and testing data sets, we used a single LC-MS 2 run to build the library and used a subsequent run from the same blood sample to search the library. In addition, for two of the species (lion and tiger), we obtained whole blood from two individuals, only one of which was used to build the database. The SDSS values were calculated for each pair of samples in the test data set and spectral libraries. The correct species most closely matched the test sample in all cases, generally with SDSS scores many fold greater than the next closest match ( Table 3 ). Even the evolutionarily most closely related pair of species in our data set (lion and tiger) were accurately identified in all cases, including samples from individuals that were not included in the database. Like all methods that depend on evolutionary relatedness, we expect to reach a limit in resolution. However, this resolution appears to be at a finer scale than between species as closely related as lions and tigers. Table 3 Evolutionary resolution. Full size table Public health efforts to control the distribution and abundance of pathogens and their vectors in nature require an accurate assessment of the factors that affect the population dynamics of these species. For example, control strategies that have focused on interrupting the transmission of B. burgdorferi in P. leucopus mice have resulted in only modest success in reducing infection prevalence in I. scapularis , and thus minimal reductions in human Lyme disease risk [41] , [42] , [43] , [44] . A likely explanation for the weak effects of mouse-targeted intervention strategies is the existence of important alternative host species [5] , [16] , [45] . Methods that rapidly and reliably identify the vertebrate species on which a disease vector previously parasitized can be used to assess the importance of each vertebrate species to the maintenance and proliferation of vector populations. Public health programs can use this knowledge of the natural ecology of the parasite to design intervention strategies that target only the appropriate host species. The methodology presented here is unlikely to provide information concerning which intervention strategies are likely to be effective. However, in multi-host parasite systems where host-targeted interventions are least likely to be practical, knowing that interventions need to target only a limited set of all potential vertebrate species increases the practicality of these public health programs. In this study, we present a non-targeted, genome-free, mass spectral searching algorithm to determine the vertebrate species from which a disease vector took their last blood meal. Using this method, the remnants of blood in blacklegged ticks were detected and correctly classified to the vertebrate species from which the tick acquired their previous blood meal in 37 out of 41 cases ( Tables 1 and 2 ). Most importantly, heavily degraded remnants of the larval blood meal in nymphal ticks that were active for 5 months or more remained detectable and were correctly classified to the vertebrate species from which the tick acquired the blood in 11 out of 14 cases ( Table 2 ). These data provide proof-of-principle validation of this method in determining the relative importance of vertebrate species as hosts for vector populations in nature. The presented method compares the entire tandem mass spectral data set derived from individual vectors to spectral reference libraries derived from the whole blood of individual species to determine the source of the blood remaining in the vector. The SDSS provides a quantitative similarity measure between two sets of spectra. Although I. scapularis ticks feed only once per life stage, empirical data suggest that the spectral matching methodology can potentially identify the sources of blood in vectors that have fed multiple times in rapid succession ( Fig. 5 ). The SDSS is also evolutionarily accurate such that the evolutionary clade of the species from which a blood meal was acquired can be identified, even if the correct species is not in the reference database. For example, the absence of an S. carolinensis spectral reference library did not prevent the identification of the source of blood in engorged larval ticks that had fed on S. carolinensis squirrels to the correct evolutionary clade, sciurid rodents, which was represented in the spectral libraries by T. striatus. ( Table 1 ). Thus, an unknown blood source can be classified to the most evolutionarily related species represented in the reference library if the true species is absent from the reference library. The evolutionary accuracy of our spectra matching methodology is perhaps not surprising, given that the spectral reference libraries can be used to accurately reconstruct the evolutionary history of vertebrate hosts ( Fig. 6 ). This finding is practically useful as it indicates that the spectral reference libraries need not necessarily contain a complete set of potential host species to identify the evolutionary clade from which a blood meal was taken. For example, there is only one marsupial in Pennsylvania, the Virginia Opossum; blood meals acquired in Pennsylvania that match to the library of any marsupial can still be identified to the Virginia Opossum by inference. It is important to note that the specificity of this methodology—the level of biological organization (order, genus, species and population) to which one can confidently identify the source of a blood meal—is dependent on the species richness of the library. Thus, adding more species to the database should permit the determination of the vertebrate source of a blood meal to a finer evolutionary resolution. We expect that our method, like any method that depends on the evolutionary changes in protein sequences, will eventually reach a limit in resolution. However, this resolution appears to be at a finer scale than the most closely related species in this study, the lion and the tiger ( Table 3 ). The spectral data set similarity algorithm correctly identified the source of the blood in 23 of the 26 moulted nymphs that had fed on either M. musculus, P. leucopus or T. striatus ( Table 2 ), even when analysed up to 6 months after moulting. The efficacy of this method may be further improved by better proteome coverage, which can be readily obtained using state-of-the-art mass spectrometers. In this study, each spectral reference library was built with two replicate LC-MS 2 runs of unfractionated blood using a quadrupole ion trap mass spectrometer, leaving considerable room to improve proteome coverage. One should also note that digestion of the blood meal is likely much faster in these experimental ticks than in natural conditions as nymphs are inactive at very low winter temperatures after their larval blood meal. As environmental conditions affect digestion in ectothermic animals [46] , [47] , the detection limit of the blood proteome from the nymphal vector may be extended further under natural field conditions. Future applications of this work to field-collected ticks with a broader range of potential host species will help to further evaluate the efficacy of this methodology under natural environmental conditions. This spectral library-based approach has several distinct theoretical advantages over traditional genome-obligated proteomic data analysis methods. On the one hand, genome sequence data are not available from the vast majority of animals that are potential sources of blood meals for haematophagous parasites, which limits the potential animal species that can be included in any study using traditional methods. On the other hand, a spectral library is essentially a record of the MS-detectable proteome, including all post-translational modifications, information that is not readily deducible from the genome sequences. Experimentally observed spectra also contain information on the true intensity of fragment ions, presence of neutral-loss fragments and other unexpected but reproducible minor ions, none of which can be predicted from sequences, leading to more accurate spectral matching. In fact, the spectral matching methodology is shown to perform better than a recently proposed sequence-based methodology that utilizes sequences of dominant blood proteins (haemoglobin subunits α and β), especially in identification of the source of blood from moulted nymphal ticks ( Table 2 and Supplementary Table S2 ). This is likely because the spectral matching methodology performs an unbiased profiling that accounts for any molecules that can be ionized and fragmented in the mass spectrometer, as opposed to restricting detection to an a priori -selected set of target peptides. Proteomic profiling methodologies should also have more discriminating power and better resolution among species, as closely related species may not be distinguishable based on the sequences of a few peptides. Moreover, experimental extraction and de novo sequencing of specific proteins is also a painstaking and error-prone process. The spectral library-based approach also has several practical advantages for blood meal analysis. First, building blood spectral libraries is much cheaper and faster than genome sequencing and is accessible to researchers without direct access to such technologies ( Supplementary Table S3 ). Second, the proposed methodology requires neither the identity nor the function of detected proteins for taxonomic identification as long as the recorded mass signal is reproducible and consistent, similar to fingerprinting methodologies using DNA (ref. 48 ). Third, it is not necessary to remove tick protein contaminants during sample preparation, as this method is robust against impurities. This is because the SDSS as defined is unaffected by unmatched spectra. Lastly, spectra are stored in their entirety and can be used in future classical proteomic studies. Hence, building spectral libraries derived from blood proteomes is a promising strategy that may be applicable to identify the vertebrate source of blood meals in the multitude of vector-borne disease systems. Although our methodology was tested in a tick vector, it may be similarly successful in many other haematophagous parasites, thereby expanding our understanding of the natural life cycle of important human pathogens and aiding in the control of vectors and vector-borne diseases. More generally, this approach can potentially be used to ‘fingerprint’ any biologically complex samples for use in medical, public health and research applications, either independently or as a complementary method to DNA-based approaches. Potential future applications include identifying tissue or cell types in clinical settings, detecting the presence and abundance of microorganisms in environmental samples, and elucidating the constituents in the human gut microbiome. Software development SpectraST (version 4.0), a tandem mass spectral library building and searching program originally developed for peptide identification [39] , [49] , was extended to incorporate unidentified spectra. Specifically, spectra imported into a library can be referenced by serial identification numbers without explicit peptide sequence identification. A consensus algorithm based solely on spectral similarity was applied to combine replicate MS 2 spectra acquired multiple times due to fragmentation of the same molecule into a consensus spectrum. This procedure is common in traditional spectral library construction and produces higher-quality spectra [50] , [51] , [52] , [53] . The numbers of spectra combined into each consensus spectrum, along with the source of the sample, were recorded. Spectra with limited information, which may cause rampant indiscriminate matching, were removed by spectral filtering. For algorithm details, please refer to Supplementary Methods . SpectraST is part of the Trans-Proteomic Pipeline suite of software, an open-source and continuously maintained tool that supports all major computer platforms and mass spectrometers [54] . Spectral libraries of whole blood Spectral reference libraries were built from LC-MS 2 analyses of whole blood from each of 24 animal species: M. musculus (lab mouse) , P. leucopus (white-footed mouse) , T. striatus (eastern chipmunk) , Ovis aries (domestic sheep) , P. leo (African lion) , P. tigris (Amur tiger) , Strix varia (barred owl) , Anas platyrhynchos (mallard) , Sturnus vulgaris (starling) , Colobus guereza (black and white Colobus) , Chelodina longicollis (snake-necked turtle) , Colubrinus loveridgei (Kenyan sand boa), Rousettus aegyptiacus (Egyptian fruit bat), Pteropus rodricensis (Rodrigues Fruit bat), Tremarctos ornatus (Andean bear), Equus africanus asinus (Poitou donkey), Nanger dama mhorr (Mhorr’s gazelle), Capra aegagrus hircus (Goat), M. rufus (red kangaroo), Corucia zebrata (prehensile-tailed skink), A. mississippiensis (American alligator), Pituophis melanoleucus (northern pine snake), Malaclemys terrapin (Northern diamondback terrapin) and Rhynchocyon petersi (giant elephant shrew). These species are representative of the major clades of land animals from which blood meals may be taken by haematophagous arthropods. Animal blood was generously donated by veterinarians at the Philadelphia Zoo or acquired from laboratory animals at the University of Pennsylvania following all animal care and use guidelines. Whole-blood samples were trypsin-digested in solution, and the resulting peptide mixtures were run on an analytical C 18 nanocapilary HPLC column (Acclaim PepMap100; DIONEX) into a LCQ-Deca XP Plus quadrupole ion trap mass spectrometer [55] , [56] , [57] . Duplicate runs were performed, and spectra acquired from each species were used to build spectral reference libraries as described above ( Fig. 1 ) and in Supplementary Methods . I. scapularis tick samples Blood-fed larval ticks ( I. scapularis ) were acquired by allowing ticks to feed to repletion on a host animal and detach naturally [16] . The larval blood meal represents the first blood meal as I. scapularis ticks feed only once at each of the three life stages (larva, nymph and adult). We experimentally infested two M. musculus mice with larval ticks purchased from Oklahoma State University. Larvae that fed to repletion and naturally detached from mice were collected, either frozen immediately ( n =5) or held at 25 °C and allowed to moult to the nymphal stage. Nymphal ticks were frozen at 1 month ( n =6), 3 months ( n =6) or 6 months ( n =6) post moult for later processing and blood meal analysis. Engorged larvae that had fed upon wild P. leucopus, T. striatus or S. carolinesis were acquired as previously described [15] . Six engorged larvae from three different P. leucopus mice and two engorged larvae from two different T. straitus chipmunks were allowed to moult and held at 25 °C for 5 months post moult before being frozen for processing and blood meal analysis. Blood meal proteome analysis Whole ticks were manually crushed in 20 μl of PBS, insoluble materials removed by centrifugation at 25,000 g at room temperature, and total protein concentrations of supernatants determined by the Bradford method (Bio-Rad). Protein extracts from engorged larvae, which are composed primarily of host blood, were run on a one-dimensional NuPAGE 4–20% Bis-Tris gel (Invitrogen, Switzerland) and proteins visualized by Coomassie Blue Staining (Bio-Rad). Each lane was cut into 20 equal-width bands, which were subjected to in-gel trypsin digestion and LC-MS 2 (refs 55 , 56 , 57 ). Total protein extracts from nymphal ticks were trypsin-digested in solution before LC-MS 2 analysis without prior gel separation. Spectral data set similarity Data obtained from LC-MS 2 analyses of tick samples were searched against the spectral reference libraries by SpectraST (version 4.0) [49] , using a precursor m/z tolerance of 1.5 Da e −1 and search parameters identical to those used for traditional spectral searching ( Fig. 1 ). The number of query spectra that matched each reference library spectrum, where a match is defined as dot product >0.7 and dot bias <0.45, were counted. For each tick, the similarity between the query spectral data set and the reference library for each species was quantified by the SDSS, given by: where SDSS(q, s) is the measure of similarity between the query data set q and the reference library s , i is an index that enumerates the spectra in the query data set, m q (i) is the number of spectra in the query data set q that matches the i th spectrum in the reference library s and r s ( i ) is the number of replicates that were combined into the i th spectrum of the reference library s . With the normalization factor of the denominator, this dot product-like function ranges from 0 (no spectral matches between the query data set and the reference library) to 1 (identical distribution of spectral counts between the query data set and the reference library). The abundance of each spectrum is taken into account to improve the discriminatory power of this function. Several alternative data set similarity functions were investigated and are presented in Supplementary Fig. S1 . The data were bootstrapped [58] to obtain a statistical measure of confidence in the identification of the source of the blood meal in each tick. For each query data set, 5,000 bootstrapped samples were generated by randomly selecting, with replacement , N MS 2 spectra from the data set, where N is the total number of MS 2 spectra in the query data set. Each bootstrapped sample was searched against each reference library, and the most similar reference library (greatest SDSS score) was recorded. The confidence in the species identified as the source of the previous blood meal is the fraction of bootstrapped samples for which the most similar reference library is derived from the correct species. This strategy quantifies the uncertainty in species identification that can occur because of the stochastic selection of peptides for fragmentation in the mass spectrometer. Estimating evolutionary divergence from spectral libraries The spectral libraries built from the whole-blood samples were used to infer phylogenetic relationships among species. The blood proteome data from each species was transformed into linear vectors representing the presence (1) or absence (0) of each library spectrum, resulting in data structures similar to restriction digest data. Bayesian phylogenies were constructed from these linear vectors in MrBayes [59] . Phylogenies were reconstructed in MrBayes using all five evolutionary models (all, noabsencesites, nopresencesites, variable and informative) originally designed for restriction digest data. Data and software availability All data used in this study, including those from LC-MS 2 analyses of the whole blood of 24 animals and of blood-fed I. scapularis samples, have been deposited at the ProteomeXchange Consortium ( http://proteomecentral.proteomexchange.org ) via the PRIDE partner repository [60] under the accession code PXD000170. The software program SpectraST is part of the Trans-Proteomic Pipeline suite. The source code is available at http://www.sourceforge.net/sashimi/ , and a one-click Windows installer is available at http://tools.proteomecenter.org/ . Instructions and documentations are available at http://tools.proteomecenter.org/wiki/index.php?title=Software:SpectraST . The software is continually maintained and upgraded. Accession codes: Data from LC-MS/MS analyses of the whole blood of 24 animals and of blood-fed I. scapularis samples have been deposited at ProteomeXchange under the accession code PXD000170. How to cite this article: Önder, Ö. et al . Identifying sources of tick blood meals using unidentified tandem mass spectral libraries. Nat. Commun. 4:1746 doi: 10.1038/ncomms2730 (2013).